Large topological Hall effect in the non-collinear phase of an antiferromagnet Non-trivial spin arrangements in magnetic materials give rise to the topological Hall effect observed in compounds with a non-centrosymmetric cubic structure hosting a skyrmion lattice, in double-exchange ferromagnets and magnetically frustrated systems. The topological Hall effect has been proposed to appear also in presence of non-coplanar spin configurations and thus might occur in an antiferromagnetic material with a highly non-collinear and non-coplanar spin structure. Particularly interesting is a material where the non-collinearity develops not immediately at the onset of antiferromagnetic order but deep in the antiferromagnetic phase. This unusual situation arises in non-cubic antiferromagnetic Mn 5 Si 3 . Here we show that a large topological Hall effect develops well below the Néel temperature as soon as the spin arrangement changes from collinear to non-collinear with decreasing temperature. We further demonstrate that the effect is not observed when the material is turned ferromagnetic by carbon doping without changing its crystal structure. Topological order is an important subject for describing novel quantum phenomena in topological insulators [1] , interacting superconducting hybrid quantum circuits [2] , protected gates for fault-tolerant quantum computing [3] and magnetic materials. In the latter, the Hall effect may show a peculiar behaviour arising from non-trivial spin arrangements. The ordinary Hall effect of a conductor in a perpendicular magnetic field is usually measured as a voltage transverse to the current. In most conductors this voltage is due to the Lorentz force acting on the charge carriers. In ferromagnetic conductors, an additional anomalous Hall effect (AHE)—for which the theories usually assume a collinear spin structure—arises from magnetization and spin–orbit interaction and is present even in zero magnetic field [4] . However, in a non-coplanar spin configuration the spin chirality κ = ∑S i ·( S k × S l ) of three magnetic moments spanning a triangle can induce a finite Berry phase and an associated fictitious magnetic field. This field generates an AHE even without spin–orbit interaction λ SO , the so-called topological Hall effect (THE) [5] , [6] . Although in many materials the spin chirality cancels, a THE has been proposed for systems with topological windings of a spin texture called skyrmions or with a non-trivial spin structure [7] . In reality, both mechanisms may play a role. A THE attributed to skyrmions has been observed in the bulk and in thin films of the helimagnets MnSi (refs 8 , 9 ), MnGe (ref. 10 ) and FeGe (refs 11 , 12 ), which all have the non-centrosymmetric cubic B20 structure. A THE associated with a topologically non-trivial spin structure was observed in double-exchange ferromagnets [5] , [13] and in the frustrated magnets with pyrochlore structure [14] , [15] . In the latter, time-reversal symmetry is macroscopically broken by the chiral spin texture, which gives rise to a spontaneous Hall effect even in zero magnetic field and in the absence of magnetic dipole long-range order [16] . Theories applied to these sytems consider the electron spin strongly coupled to the localized magnetic moments. In the weak-coupling regime, chirality and spin–orbit interaction have been taken into account perturbatively including metallic spin glasses with random chiral order [17] . A chirality-driven Hall effect might be present in reentrant spin glasses where the AHE due to λ SO appears in the ferromagnetic regime while in the spin-glass regime the additional chirality contribution sets in due to spin canting. A chirality mechanism was also proposed for non-coplanar cubic antiferromagnets with a distorted lattice [18] . In the cubic heavy-fermion metal UCu 5 with localized 5f moments a large geometrical Hall effect has been attributed to frustration-induced magnetic order without assuming spin–orbit scattering [19] . This suggests that a THE might also appear in non-cubic antiferromagnets with a non-trivial spin structure. In this respect, antiferromagnetic Mn compounds are potential candidates because the Mn 3d magnetic moments are very susceptible to their local environment and nearest-neighbour interactions giving rise to different local Mn moments. Recently, it has been pointed out that an AHE can arise in a non-collinear antiferromagnet motivating the investigation of a material with collinear and non-collinear antiferromagnetic phases at different temperatures [20] . This unusual situation arises in orthorhombically distorted hexagonal Mn 5 Si 3 . The intermetallic compound Mn 5 Si 3 with hexagonal D8 8 structure has been investigated in detail by neutron scattering [21] , [22] , [23] , [24] . In the paramagnetic state, the unit cell (space group P6 3 /mcm) contains Mn 1 and Mn 2 atoms on two inequivalent lattice sites. The occurrence of long-range antiferromagnetic order below the Néel temperature T N2 =99 K is accompanied by an orthorhombic distortion. In the AF2 phase between T N2 and T N1 =66 K, the Mn 1 and one-third of the Mn 2 atoms do not exhibit an ordered magnetic moment. The remaining Mn 2 atoms have moments oriented parallel and antiparallel to the crystallographic b axis in a collinear fashion [22] , [23] , see Fig. 1a and Supplementary Movie 1 . 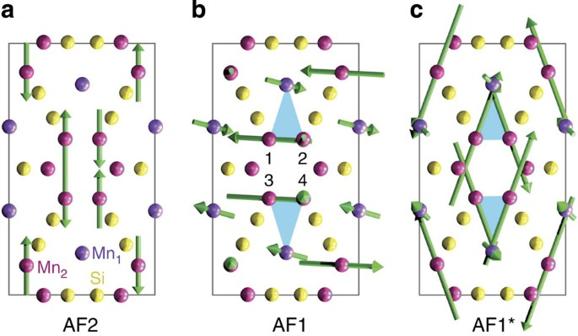Figure 1: Magnetic structure of Mn5Si3. (View along the crystallographiccaxis). (a) Collinear AF2 phase according to refs22,23. (b) Non-collinear AF1 phase according to ref.21. (c) Non-collinear AF1* phase according to ref.23. Violet: Mn1, magenta: Mn2, yellow: Si. Solid lines indicate the orthorhombic unit cell. The length of each arrow indicates the size of the local magnetic moment projected to the plane of view (arrow length inacorresponds to a magnetic moment of 1.5μB). While arrows 1 and 3 are aligned almost in the plane, arrows 2 and 4 are pointing downwards and upwards, respectively, perpendicularly to the plane. Blue triangles exemplarily show the triangular spin arrangements formed by moments Mn1and Mn2. For a three-dimensional (3D) view of the structure see theSupplementary Movies 1–3. Figure 1: Magnetic structure of Mn 5 Si 3 . (View along the crystallographic c axis). ( a ) Collinear AF2 phase according to refs 22 , 23 . ( b ) Non-collinear AF1 phase according to ref. 21 . ( c ) Non-collinear AF1* phase according to ref. 23 . Violet: Mn 1 , magenta: Mn 2 , yellow: Si. Solid lines indicate the orthorhombic unit cell. The length of each arrow indicates the size of the local magnetic moment projected to the plane of view (arrow length in a corresponds to a magnetic moment of 1.5 μ B ). While arrows 1 and 3 are aligned almost in the plane, arrows 2 and 4 are pointing downwards and upwards, respectively, perpendicularly to the plane. Blue triangles exemplarily show the triangular spin arrangements formed by moments Mn 1 and Mn 2 . For a three-dimensional (3D) view of the structure see the Supplementary Movies 1–3 . Full size image In the low-temperature antiferromagnetic AF1 phase below T N1 the magnetic structure has monoclinic symmetry with atomic positions that can described with orthorhombic symmetry of the Ccmm space group without inversion symmetry [21] , [23] , [24] . In this phase, the Mn 1 atoms acquire a moment, in addition to realigned Mn 2 moments. The moments point into different directions forming a highly non-collinear antiferromagnetic structure ( Fig. 1b ). One-third of the Mn 2 atoms still do not exhibit an ordered magnetic moment. The non-collinearity is attributed to topological frustration [21] , [24] . Recently, T N2 and T N1 have been determined from susceptibility measurements [23] . For T < T N1 a non-collinear phase has been suggested as well, however with a different spin arrangement, which we denote AF1* ( Fig. 1c ). Both arrangements AF1 and AF1* have in common that the Mn 1 atoms exhibit an ordered moment only below T N1 , causing non-collinearity with a non-zero spin chirality for each triangular spin arrangement, see Fig. 1b,c and Supplementary Movies 2 and 3 . The nuclear/magnetic structure in the AF1/AF1* phase can be modified by a magnetic field from monoclinic to orthorhombic symmetry, thereby strengthening the AF2 arrangement. In a magnetic field the sample is already in the AF2 phase at T (1T)=63 K and at T (3.6T)=58 K (ref. 24 ). In 4T the orthorhombic phase remains down to T =5 K (ref. 23 ). In contrast to antiferromagnetic Mn 5 Si 3 , the isostructural carbon-doped Mn 5 Si 3 C x shows ferromagnetic order with a maximum Curie temperature T C =352 K for x =0.8 (refs 25 , 26 ). A similar doping effect was observed in isostructural Mn 5 Ge 3 C x thin films with T C =430–450 K ( x =0.7–0.8) much higher than for Mn 5 Ge 3 (refs 27 , 28 ), where the enhanced ferromagnetic stability was attributed to a carbon-mediated 90° superexchange between Mn atoms mediated by carbon [29] . In Mn 5 Ge 3 non-collinearity may be stabilized by uniaxial distortion [30] . Hence, the carbon-induced change of magnetic order provides a unique opportunity to compare the AHE of isostructural antiferromagnetic Mn 5 Si 3 and ferromagnetic Mn 5 Si 3 C 0.8 . For this purpose, here we measure the Hall effect ρ xy ( H , T ), the magnetoresistance (MR) ρ xx ( H , T ) and the magnetization M ( H , T ) for various magnetic fields H and temperatures T to separate the ordinary and anomalous contributions to the Hall effect. We observe an additional contribution to the anomalous Hall effect in the non-collinear regime of antiferromagnetic Mn 5 Si 3 , which we propose to be of topological origin. This contribution is not observed in the collinear antiferromagnetic regime of Mn 5 Si 3 and is also absent in Mn 5 Si 3 C 0.8 , that is, when the material is turned ferromagnetic by carbon doping without changing its crystal structure. The results motivate further search for the observation of a THE in other antiferromagnets with a non-trivial spin structure, thus widening considerably the arena of materials suitable for exploiting the THE in the future. 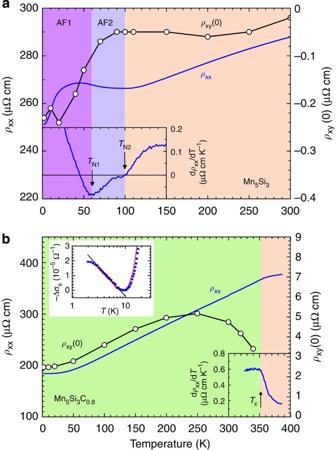Figure 2: Temperature dependence of the resistivity. Longitudinal resistivityρxx(solid line) and Hall resistivityρxy(0) extrapolated toH=0 for 45-nm-thick films of (a) antiferromagnetic Mn5Si3and (b) ferromagnetic Mn5Si3C0.8. Lower insets show the kinks in dρxx(T)/dTin the vicinity of the magnetic transition temperatures. The upper inset inbshows a semilogarithmic plot of the variation of the sheet conductance, where the solid line indicates a behaviour −Δσs(T)∝log(T/8 K). Resistivity Figure 2a shows the temperature dependence of the resistivity ρ xx of a 45-nm antiferromagnetic Mn 5 Si 3 film. Below T N2 =100 K, the deviation from the roughly linear dependence observed at high temperatures indicates the onset of antiferromagnetic order with a shallow minimum of ρ xx at T N2 and a broad maximum below T N2 . For lower temperatures T << T N1 , the observed ρ xx ∝ T 2 behaviour is attributed to the scattering of electrons by antiferromagnetic spin waves [31] , [32] . Similar behaviour has been observed in Mn 5 Si 3 polycrystals [33] , single crystals [34] and thin films, and has been discussed in detail [31] . The two magnetic phase transitions are clearly resolved as kinks in the derivative d ρ xx ( T )/d T at T N1 ( ρ xx )≈60 K and T N2 ( ρ xx )≈100 K, see Fig. 2a inset. T N2 ( ρ xx ) and T N1 ( ρ xx ) are in good agreement with values obtained from neutron diffraction [21] , [22] , [23] , [24] , [35] and from thermal expansion [36] . Figure 2: Temperature dependence of the resistivity. Longitudinal resistivity ρ xx (solid line) and Hall resistivity ρ xy (0) extrapolated to H =0 for 45-nm-thick films of ( a ) antiferromagnetic Mn 5 Si 3 and ( b ) ferromagnetic Mn 5 Si 3 C 0.8 . Lower insets show the kinks in d ρ x x ( T )/d T in the vicinity of the magnetic transition temperatures. The upper inset in b shows a semilogarithmic plot of the variation of the sheet conductance , where the solid line indicates a behaviour −Δσ s ( T ) ∝ log( T /8 K). Full size image The ρ xx ( T ) behaviour of the 45-nm ferromagnetic Mn 5 Si 3 C 0.8 film at low temperatures ( Fig. 2b ) is in agreement with earlier data, including a logarithmic T dependence of the sheet conductance ( Fig. 2b upper inset) attributed to the scattering of conduction electrons by two-level systems with a crossover to Fermi-liquid behaviour below ≈1 K (ref. 31 ). At high temperatures, the slope of ρ xx ( T ) changes at the Curie temperature T C =352 K. This is again resolved more clearly in the derivative dρ xx ( T )/ dT ( Fig. 2b lower inset) where a kink occurs at the critical temperature T C (ref. 37 ). T C is in very good agreement with data published earlier for optimally carbon-doped Mn 5 Si 3 C 0.8 (refs 26 , 31 ). Magnetoresistance The MR ρ xx ( H ⊥ )− ρ xx (0) of both samples shown in Fig. 3 is negative for all temperatures and does not saturate. Hence, a positive contribution from the orbital motion of charge carriers affected by the Lorentz force is of minor importance. The MR ratio at 8 T, ( ρ x x (8 T)− ρ xx (0))/ ρ xx (0), strongly varies with temperature. The inset of Fig. 3a shows that the MR ratio of Mn 5 Si 3 in the AF1 phase first decreases and then increases with increasing T until it becomes almost zero in the paramagnetic phase for T > T N2 . 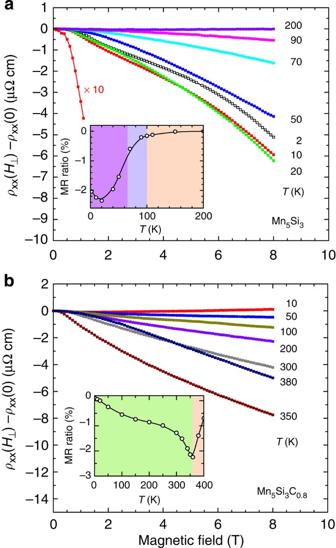Figure 3: Magnetoresistance. ρxxin perpendicular magnetic fieldHat various temperaturesTfor (a) antiferromagnetic Mn5Si3and (b) ferromagnetic Mn5Si3C0.8. Insets show the temperature dependence of the MR ratio (ρxx(8 T)−ρxx(0))/ρxx(0). Figure 3: Magnetoresistance. ρ xx in perpendicular magnetic field H at various temperatures T for ( a ) antiferromagnetic Mn 5 Si 3 and ( b ) ferromagnetic Mn 5 Si 3 C 0.8 . Insets show the temperature dependence of the MR ratio ( ρ xx (8 T)− ρ xx (0))/ ρ xx (0). Full size image The MR of weak metallic antiferromagnets with itinerant s and d electrons, as exemplified by a number of Mn alloys, has been studied theoretically in a model where s electrons from the conduction band are scattered by spin-density fluctuations [38] . In a field perpendicular to the sublattice magnetization, a negative MR ∝ − H 2 for weak fields, followed by a linear behaviour is expected for all temperatures. This expectation qualitatively agrees with the MR behaviour of Mn 5 Si 3 , cf . the data for T =10 K in Fig. 3a . In a field parallel to the sublattice magnetization, a positive MR is expected close to the field H sf where a spin-flop transition occurs. In Mn 5 Si 3 , H sf corresponds to the metamagnetic-transition field, which is larger than 8T for T <60 K in single crystals and is obviously not reached in the present measurements on polycrystalline films [34] . A different temperature dependence of the MR ratio is observed for ferromagnetic Mn 5 Si 3 C 0.8 ( Fig. 3b , inset). Here the MR ratio decreases with increasing temperature all the way up to the Curie temperature T C and increases again with a distinct minimum at T C . The negative MR in perpendicular field was reported earlier [31] and was attributed to the damping of spin waves by the magnetic field leading to a decrease of the scattering of electrons by spin waves [39] . Magnetization The magnetization of antiferromagnetic Mn 5 Si 3 ( Fig. 4a ) increases with increasing field with a small negative curvature and does not saturate in our maximum field of 5 T. The absolute value of M at μ 0 H =5 T roughly agrees with M determined for Mn 5 Si 3 single crystals for T > T N1 (ref. 34 ). A field-induced transition from the low-temperature non-collinear phase to a phase akin to the high-temperature collinear phase reported for the single crystals [34] is not visble in M ( H ) of the polycrystalline film in perpendicular magnetic field. However, we emphasize that T N1 is clearly observed in d ρ xx ( T )/d T ( Fig. 2a inset) and the static susceptibility M / H versus T exhibits a broad maximum around the Néel temperatures, which is best observed for small μ 0 H =10 mT and shifts toward lower T with increasing field, see Fig. 4a inset. This is in agreement with recent measurements of the dc susceptibility χ ( T ), which show a jump of χ ( T ) at T N1 but only a shallow kink at T N2 (ref. 23 ). 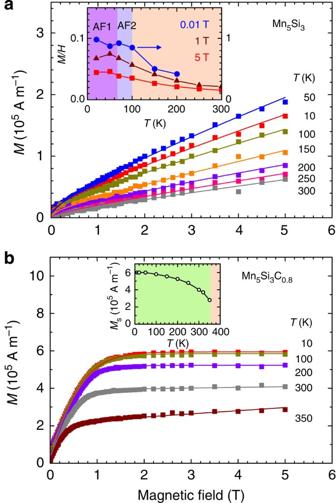Figure 4: Magnetization. M(H) in perpendicular magnetic fieldHat various temperaturesTfor (a) antiferromagnetic Mn5Si3and (b) ferromagnetic Mn5Si3C0.8. Inset inashowsM(T)/Hfor different magnetic fields, inset inbshows the saturation magnetizationMS(T). Figure 4: Magnetization. M ( H ) in perpendicular magnetic field H at various temperatures T for ( a ) antiferromagnetic Mn 5 Si 3 and ( b ) ferromagnetic Mn 5 Si 3 C 0.8 . Inset in a shows M ( T )/ H for different magnetic fields, inset in b shows the saturation magnetization M S ( T ). Full size image M ( H ) of ferromagnetic Mn 5 Si 3 C 0.8 shows a hard-axis behaviour without hysteresis due to the strong shape anisotropy of the thin film in a perpendicular magnetic field (see Fig. 4b ). The saturation magnetization M S ( T ) determined at μ 0 H =6T shows the characteristic dependence of a ferromagnet with M S (10 K)=6 × 10 5 A −1 m −1 corresponding to a magnetic moment of 1.3 μ B per Mn, somewhat higher than observed earlier for 100-nm Mn 5 Si 3 C 0.8 films [31] . Hall effect The Hall resistivity ρ xy ( H ) of antiferromagnetic Mn 5 Si 3 shown in Fig. 5a is strongly non-linear and shows a positive curvature at low fields and a roughly linear behaviour at high fields without saturation. For clarity, only a subset of data is shown. The Hall resistivity ρ xy (0) at zero magnetic field is obtained by linear extrapolation of the high-field data in the field interval 5–8 T to H =0. The temperature dependence of ρ xy (0) ( Fig. 2a ) strongly deviates from ρ xx ( T ) and does not allow a simple scaling of ρ xy ( ρ xx ) [40] . ρ xy (0) is almost zero above T N2 and strongly decreases to negative values well below T N2 . This is in qualitative agreement with theory predicting a vanishing Berry curvature and zero-field Hall conductivity in the paramagnetic and collinear antiferromagnetic phases, while a large AHE is expected to appear in the non-collinear antiferromagnetic phase [20] . 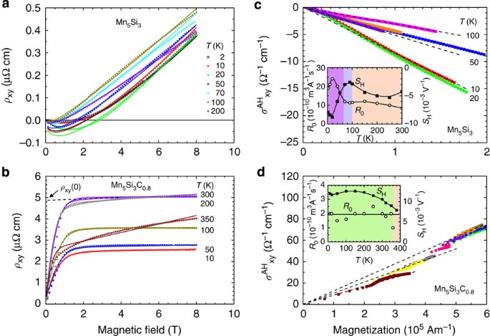Figure 5: Hall effect and anomalous Hall conductivity. (a,b) Hall resistivityρxy(H) for various temperaturesT. Solid lines show fits according to Eqn. 1 to measured data (symbols). Dashed line inbshows the linear extrapolation of the high-field data in the field interval 5–8 T toH=0 yieldingρxy(0). (c,d) Anomalous contributionto the Hall conductivity for various temperaturesT. Dashed lines indicate a linear behaviour. Insets show the temperature dependence of the ordinary Hall coefficientR0and of the anomalous Hall coefficientSH. Figure 5: Hall effect and anomalous Hall conductivity. ( a , b ) Hall resistivity ρ xy ( H ) for various temperatures T . Solid lines show fits according to Eqn. 1 to measured data (symbols). Dashed line in b shows the linear extrapolation of the high-field data in the field interval 5–8 T to H =0 yielding ρ xy (0). ( c , d ) Anomalous contribution to the Hall conductivity for various temperatures T . Dashed lines indicate a linear behaviour . Insets show the temperature dependence of the ordinary Hall coefficient R 0 and of the anomalous Hall coefficient S H . Full size image Figure 5b shows the Hall resistivity ρ xy ( H ) of ferromagnetic Mn 5 Si 3 C 0.8 . The steep increase at low fields and a leveling-off towards saturation at high fields resembles the magnetization behaviour M ( H ) in Fig. 4b . Furthermore, ρ xy (0) shows a low-temperature behaviour similar to ρ xx ( T ) ( Fig. 2b ) and decreases towards zero for T approaching T C due to the strong decrease of the magnetization M ( T ). In general, the Hall resistivity ρ xy = R 0 B + R S μ 0 M comprises the ordinary term and the anomalous term due to the magnetization M (ref. 4 ). R 0 =( e n eff ) −1 and R S are the ordinary and anomalous Hall coefficients, respectively, where n eff is the effective carrier density that depends on the scattering rates in the case of carriers in multiple bands. μ 0 the magnetic constant, M the magnetization and B = μ 0 ( H + M (1− N )), where the demagnetization factor N for thin films in a perpendicular magnetic field is N ≈1. Hence, B = μ 0 H and the Hall resistivity and Hall conductivity can be written as where and we have assumed ρ xy << ρ xx . These equations have been applied previously to uncover the THE in the helimagnets MnSi (ref. 8 ), MnGe (ref 10 ) and FeGe (ref 12 ). They are valid in a weak magnetic field for which ω c τ <<1, where ω c = eB / m is the cyclotron frequency, τ = m / ne 2 ρ xx is the electron scattering time and m is the electron mass. In the present case, this condition is fulfilled up to the maximum applied field of 8 T for which we obtain ω c τ = BR 0 / ρ xx =0.004. The AHE in general depends on the resistivity ρ xx and contains an intrinsic contribution originating from the Berry-phase-curvature correction to the group velocity of a Bloch electron induced by spin–orbit interaction as well as extrinsic contributions arising from a side-jump mechanism and skew scattering ( ∝ ρ xx ) [4] . A scaling relation has been proposed to describe the behaviour in the different transport regimes [41] . The conventional theories of the AHE in ferromagnets derived via pertubation theory often consider that S H is proportional to the spin–orbit interaction and independent of temperature below the Curie temperature T C (refs 4 , 42 ). We separate the different contributions to the Hall effect by application of equations 1 and 2 (refs 40 , 43 , 44 , 45 , 46 ). Figure 5c,d shows versus M for different T for the two compounds. For clarity, again only a subset of data is shown. R 0 was used as a free parameter with the constraint of a proportionality between and M , that is, as reported earlier for Mn 5 Ge 3 (ref. 43 ). The influence of the MR on the Hall effect cancels by this procedure and we obtain the Hall coefficients R 0 and S H plotted in Fig. 5c,d (insets). Similar values can be obtained from a plot ρ xy / μ 0 H versus as done previously for MnSi (ref. 46 ). For antiferromagnetic Mn 5 Si 3 , a positive R 0 and a negative S H are obtained. The former indicates hole-like conduction. Furthermore, while both coefficients are independent of temperature for T > T N1 , in particular in the AF2 phase between T N1 and T N2 , their values vary strongly for T < T N1 with a maximum of R 0 ( T ) and a minimum of S H ( T ) around 10–20 K, see Fig. 5c (inset). For T > T N1 , R 0 ≈10 −9 m 3 A −1 s −1 corresponds to an effective carrier density n eff =6 × 10 21 holes cm −3 , whereas at low T , n eff is reduced to 3 × 10 21 holes cm −3 . The strong variation of both coefficients below T N1 is possibly due to the interplay of magnetic order and electronic transport. A similar correlation of R 0 and S H has been reported for stoichiometric NbFe 2 in the spin-density-wave regime where R 0 >0 has a minimum above T N and increases at low T , while S H <0 has a minimum at T N (ref. 46 ). The minimum of R 0 was tentatively attributed to a change in the relative scattering of the two conduction bands. The calculated ρ xy ( H ) values in Fig. 5a (solid lines) are in good agreement with the measured Hall resistivities for temperatures T ≥70 K, that is, in the collinear antiferromagnetic AF2 phase and in the paramagnetic phase. In contrast, in the non-collinear phase at low magnetic fields and temperatures T <70 K the data show a strong enhancement of the measured ρ xy compared with the calculated values (solid lines) below 3 T, see the replotted data in Fig. 6a . Adding a contribution ∝ ρ xx to the AHE arising from skew scattering does not reduce the difference because the Hall effect of the highly resistive films is dominated by contributions (refs 4 , 41 ). The strong enhancement of ρ xy at low fields is observed even more clearly for a thicker film of 160 nm thickness ( Fig. 6b ), which has a lower residual resistivity ρ xx (2 K)=161 μΩ cm. For temperatures T << T N1 and below a critical field H c indicated by arrows, the experimental ρ xy ( H ) data strongly deviate from the roughly linear high-field behaviour. For both films, the additional contribution to ρ xy (yellow area) is of similar size. 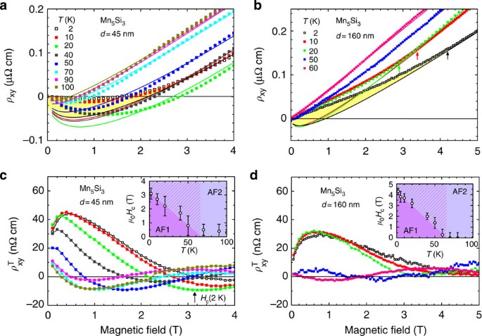Figure 6:Topological Hall effect in Mn5Si3. (a)ρxyof a 45-nm-thick film for small magnetic fieldsH,cf.Fig. 5a. (b)ρxyof a 160 nm-thick film. (c,d)for various temperaturesT. Inset shows the temperature dependence ofHcindicated in the main panel forT=2 K. Arrows indicate the fieldHcbelow whichρxydeviates from the high-field behaviour. Yellow areas inaandbvisualise the additional contribution arising from the THE atT=2 K. Error bars in the insets indicate the uncertainty in the determination ofHcdue to variation ofaround zero at high fields (±5 nΩcm ford=45 nm, ±3 nΩcm ford=160 nm). Figure 6: Topological Hall effect in Mn 5 Si 3 . ( a ) ρ xy of a 45-nm-thick film for small magnetic fields H , cf . Fig. 5a . ( b ) ρ xy of a 160 nm-thick film. ( c , d ) for various temperatures T . Inset shows the temperature dependence of H c indicated in the main panel for T =2 K. Arrows indicate the field H c below which ρ xy deviates from the high-field behaviour. Yellow areas in a and b visualise the additional contribution arising from the THE at T =2 K. Error bars in the insets indicate the uncertainty in the determination of H c due to variation of around zero at high fields (±5 nΩcm for d =45 nm, ±3 nΩcm for d =160 nm). Full size image Figure 6c,d shows the additional contribution to the AHE determined by . For both samples, is positive with a broad maximum of similar magnitude at low fields and decreases with increasing temperature until it vanishes at T ≈70 K. At our lowest temperature T =2 K and at a field below 3–4 T the large completely compensates the AHE, cf . Fig. 6a,b . The temperature dependence of the critical field H c above which ρ xy follows the high-field behaviour (Eqn. 1) and is reduced to zero is shown in the insets of Fig. 6c,d . Hence, measurement of the Hall effect allows to establish the magnetic-field-induced phase diagram of the AF1 phase of antiferromagnetic Mn 5 Si 3 with a linear dependence H c ( T )≈ H c (0)(1− T / T N1 ). The behaviour of in Fig. 6c,d suggests that the non-collinear magnetic structure is gradually weakened upon approaching the phase boundary. In contrast to antiferromagnetic Mn 5 Si 3 , for ferromagnetic Mn 5 Si 3 C 0.8 both coefficients R 0 and S H are positive ( Fig. 5d , inset) and the calculated ρ xy values (Eqn. 1) shown as solid lines in Fig. 5b are in good agreement with the measured data. R 0 ≈2 × 10 −10 m 3 A −1 s −1 is independent of temperature and corresponds to n eff =3 × 10 22 holes cm −3 , that is, a factor five higher than for Mn 5 Si 3 , suggesting p-type doping by carbon. This can be due to a carbon-induced change of the electronic band structure and an increased density of states at the Fermi level, similar to what has been found for Mn 5 Ge 3 C x (ref. 29 ). A confirmation of this conjecture has to await band-structure calculations for Mn 5 Si 3 C x . S H is roughly independent of temperature up to ≈200 K and only gradually decreases for temperatures close to T C . A finite S H is observed even in the paramagnetic regime above T C similar to Mn 5 Si 3 , arising from the temperature-independent spin–orbit interaction, which we estimate to be λ SO ≈100 μeV for Mn 5 Si 3 C 0.8 (refs 5 , 17 , 42 ). In Mn 5 Si 3 , the different Mn moments located at inequivalent lattice sites are susceptible to magnetic frustration yielding below T N1 a highly non-collinear spin structure AF1 (or AF1*) in contrast to the collinear antiferromagnetic structure AF2 above T N1 . The chirality in the AF2 phase of collinearly arranged Mn 2 moments is zero. In the AF1 phase, the Mn 2 rotate away from their collinear orientation and, in addition, the Mn 1 atoms acquire an ordered moment resulting in a triangular non-collinear and non-coplanar arrangement of magnetic moments with a finite chirality below T N1 . This gives rise to an additional contribution to the AHE, which we propose to be of topological origin. This topological Hall effect explains the deviation of the measured data from the calculated ρ xy ( H ) curves. The absolute magnitude of the maximum of is comparable to the THE of polycrystalline MnGe films [10] and of sputtered FeGe films [12] . is independent of temperature below T ≤20 K<< T N1 , which supports our assignment of this feature to a THE. For a magnetic field H > H c the non-collinear spin structure associated with the THE disappears. Remarkably, we observe a roughly linear decrease of H c with T crossing the abcissa at T ≈ T N1 where the Mn 1 moments lose their magnetic moment and the Mn 2 moments reorientate in a collinear fashion. This strongly suggests that indeed arises from a THE due to the non-collinear and non-centrosymmetric magnetic structure in the AF1 phase, which is reduced by an applied field leading to a collinear alignment of moments. A scenario based on chirality also explains the opposite signs of S H and R 0 . In the presence of a non-trivial spin structure, the internal field due to chirality acts to cancel the applied field implying opposite signs for S H and R S (ref. 5 ). As already mentioned, in Mn 5 Si 3 single crystals application of a magnetic field at T < T N1 can change the magnetic structure from monoclinic to orthorhombic and induce a collinear alignment of the moments similar to the AF2 phase [23] . The boundary between the AF1 phase and the field-induced AF2 phase represented by H c ( T ) is in very good agreement with the results from neutron scattering. In μ 0 H =4 T the orthorhombic symmetry was observed down to 5 K (ref. 23 ) and in μ 0 H =1 T it was still observed at 63 K (ref. 24 ). This agreement provides strong additional evidence that the origin of is a THE in the AF1 phase due to the non-collinear magnetic structure that disappears as soon as the moments get aligned by the field. This is qualitatively different from the large geometrical Hall effect in the cubic heavy-fermion system UCu 5 , where the anomaly of ρ xy in the magnetically frustrated phase diminishes at a magnetic field of ≈7 T, independent of temperature [19] . In this case, the progression of a magnetically frustrated 4- q phase below T 2 =1.2 K and a coplanar 1- q phase above T 2 has been inferred from detailed magnetization and resistivity measurements. The resulting phase diagram is different from the phase diagram proposed in previous reports [47] , [48] . Finally, our measurements on ferromagnetic Mn 5 Si 3 C 0.8 do not show any evidence for an additional contribution to the AHE arising from a THE. The temperature-independent Hall coefficients R 0 and S H and the linear ρ xx ( T ) behaviour support the classification of Mn 5 Si 3 C 0.8 as a metallic ferromagnet. This is in line with previous investigations [31] , [49] and presumably originates from superexchange between Mn 2 moments via carbon as reported for Mn 5 Ge 3 C x (ref. 29 ). This supports our conclusion that the additional contribution to the AHE attributed to a THE in antiferromagnetic Mn 5 Si 3 arises from the non-collinear magnetic structure in the AF1 phase. Film growth and structural characterization Polycrystalline films of thickness d =45 nm and 160 nm of Mn 5 Si 3 and d =45 nm of Mn 5 Si 3 C 0.8 were prepared by magnetron sputtering under Ar atmosphere ( p Ar =0.8 Pa) in a vacuum system with a base pressure P <10 −4 Pa. Mn, Si, Ge and C were sputtered from elemental targets onto -oriented sapphire substrates (thickness 0.53 mm) at a substrate temperature T S =470 °C and were characterized by X-ray diffraction to confirm formation of the Mn 5 Si 3 -type structure [26] , [31] . The films have a coarsely grained morphology with an average grain size equal to the film thickness [31] . For the resistivity measurements, the substrate was covered by a mechanical mask to obtain a Hall-bar layout. Resistivity measurements Resistivities were measured between 2 and 400 K in a 4 He cryostat of a physical property measuring system (PPMS, Quantum Design) equipped with a superconducting solenoid providing magnetic fields up to 9 T. The longitudinal resistivity ρ xx = V x wd / LI x was determined from the longitudinal voltage V x measured along a stripe of length L =8 mm in x direction and width w =0.5 mm with current I x (four-probe method). The Hall effect was measured as transverse voltage V y to the current I x in perpendicular magnetic field H , where the Hall resistivity was measured via ρ xy = V y d / I x for positive and negative magnetic fields and the total Hall resistivity was determined by ρ xy ( H )=( ρ xy (+ H )− ρ xy (− H ))/2. Magnetization measurements The magnetic moment of the samples was measured in a superconducting quantum-interference device (SQUID) magnetometer (Quantum Design) between 10 and 350 K for magnetic fields up to 5 T. The magnetization M of the films was determined by subtracting the diamagnetic signal of the Al 2 O 3 substrate from the raw data. For this purpose the magnetic susceptibility χ ( T )= M / H of Al 2 O 3 was determined from the linear behaviour of the magnetization M ( H ) above the saturation field for Fe films deposited on Al 2 O 3 . χ ( T ) smoothly decreases between −16.27 ( T =10 K) and −16.87 ( T ≥150 K) and is in good agreement with data reported by Smith et al. [50] How to cite this article: Sürgers, C. et al. Large topological Hall effect in the non-collinear phase of an antiferromagnet. Nat. Commun. 5:3400 doi: 10.1038/ncomms4400 (2014).